Spontaneous chiral symmetry breaking in metamaterials Spontaneous chiral symmetry breaking underpins a variety of areas such as subatomic physics and biochemistry, and leads to an impressive range of fundamental phenomena. Here we show that this prominent effect is now available in artificial electromagnetic systems, enabled by the advent of magnetoelastic metamaterials where a mechanical degree of freedom leads to a rich variety of strong nonlinear effects such as bistability and self-oscillations. We report spontaneous symmetry breaking in torsional chiral magnetoelastic structures where two or more meta-molecules with opposite handedness are electromagnetically coupled, modifying the system stability. Importantly, we show that chiral symmetry breaking can be found in the stationary response of the system, and the effect is successfully demonstrated in a microwave pump-probe experiment. Such symmetry breaking can lead to a giant nonlinear polarization change, energy localization and mode splitting, which provides a new possibility for creating an artificial phase transition in metamaterials, analogous to that in ferrimagnetic domains. Symmetry is an important concept in modern physics that describes the invariance of geometries or laws under specified transformations. Despite the beauty of symmetry, broken symmetry has been shown to play a significant role in the existence of new phenomena in various systems. In general, symmetry breaking can be divided into two types: explicit symmetry breaking and spontaneous symmetry breaking. The former indicates that the dynamic equations of a system are not invariant under the specified symmetry group; this can be achieved by introducing additional terms that manifestly break the original symmetry. The latter effect, in contrast, is a spontaneous process, during which a system in an initially symmetric state ends up in an asymmetric state, even though the underlying dynamic equations are still invariant under a symmetry transformation [1] , [2] . Spontaneous symmetry breaking is an underlying mechanism of many fundamental phenomena. Well-known examples include spontaneous magnetization [3] , the symmetry breaking in strong interaction that is responsible for the bulk of mass of nucleons [4] , [5] , the recently discovered Higgs boson [6] , [7] , [8] , [9] , [10] and the breaking of chiral symmetry in biochemistry that is crucially important for the homochirality of biomolecules [11] , [12] , [13] . Recent studies of spontaneous symmetry breaking in nonlinear optical systems [14] , [15] , [16] and Bose–Einstein condensates [17] , [18] further underline its ubiquity. In the field of metamaterials, the introduction of structural asymmetry provides additional degrees of freedom in controlling light-matter interaction. A variety of phenomena, including Fano resonances [19] , [20] and directive in-plane scattering [21] , [22] , [23] , [24] , [25] , can be obtained via the reduced mirror symmetry of a system. Complete breaking of mirror symmetry can result in optical activity [26] , [27] , [28] , circular dichroism [29] , [30] and asymmetric transmission [31] , [32] , which have been extensively studied in the context of chiral metamaterials. These scenarios can all be classified as explicit symmetry breaking, since asymmetry is artificially introduced into the Hamiltonian by modifying the configuration of the system. On the other hand, nonlinear metamaterials [33] , [34] provide a unique platform for the study of spontaneous symmetry breaking. Various nonlinear localization effects such as solitons [35] , [36] , [37] and domain walls [38] , [39] have been studied theoretically, in particular in the context of metamaterials with nonlinear inclusions such as varactor diodes [40] . Recently, the concept of magnetoelastic metamaterials was introduced to describe a new generation of nonlinear metamaterials [41] . The nonlinear response in these structures originates from the coupling between electromagnetic (EM) resonances and elastic deformation of the structure, rather than a local change of the EM environment. This idea was later extended to chiral metamaterials by exploiting torsion [42] or structural compression [43] , and a rich variety of strong nonlinear responses such as large self-tuning, bistability [42] , [44] , damping-immune self-oscillation and dynamic optical activity [45] were shown to be feasible under moderate pump powers. In this paper, we study the nonlinear behaviour when two or more torsional meta-molecules with opposite handedness (the so-called metamaterial enantiomers) are electromagnetically coupled (see Fig. 1 ). The term ‘chiral symmetry’ here follows the same definition as in previous studies of enantiomeric molecules [46] , [47] —for a given set of dynamic equations F that describe the interaction and evolution of the metamaterial enantiomers ( x L , x R ), they are covariant under parity transformation P , that is, P [ F ( x L , x R )]= F ( x R , x L ). Intuitively, under such a symmetry condition, torsional meta-molecules with opposite handedness should have identical magnitudes of EM response if they are equally excited; the net chirality of the whole system should also vanish due to chiral symmetry. However, our study explicitly shows that when the interaction between meta-molecules becomes sufficiently strong, the system undergoes spontaneous symmetry breaking and becomes chiral. 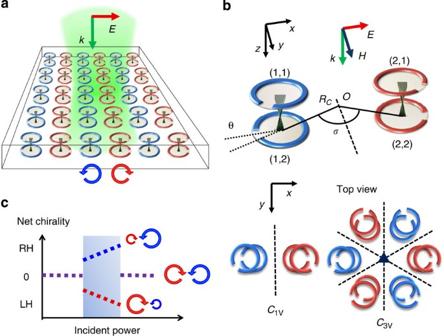Figure 1: Schematics of torsional metamaterial enantiomers and spontaneous chiral symmetry breaking. (a) Conceptual layout of torsional metamaterials with chiral symmetry. Each meta-molecule consists of two coaxial twisted meta-atoms (SRRs) connected elastically, and meta-molecules with right and left handedness are plotted in blue and red colours, respectively. The green-shaded region represents the incident EM waves, and the responses of enantiomers are denoted by circular arrows. (b) Configurations of enantiomeric meta-molecules withCNvsymmetry. The displacement vector between a meta-molecule and the rotation centreOisRCand the rotation angleσ=π/N.θl,jis the twist angle of an SRR with respect toRC, where the first index reflects the number of SRR pair, and the second index distinguishes between the upper (j=1) and lower (j=2) SRRs in the pair. The dashed lines are the axes of mirror symmetry. (c) Schematic showing the phase transition of net chirality of the system when the incident power changes. In the shaded regime, spontaneous chiral symmetry breaking occurs and the net chirality can fall into either the left-handed (LH) or the right-handed (RH) regime. Figure 1: Schematics of torsional metamaterial enantiomers and spontaneous chiral symmetry breaking. ( a ) Conceptual layout of torsional metamaterials with chiral symmetry. Each meta-molecule consists of two coaxial twisted meta-atoms (SRRs) connected elastically, and meta-molecules with right and left handedness are plotted in blue and red colours, respectively. The green-shaded region represents the incident EM waves, and the responses of enantiomers are denoted by circular arrows. ( b ) Configurations of enantiomeric meta-molecules with C N v symmetry. The displacement vector between a meta-molecule and the rotation centre O is R C and the rotation angle σ = π / N . θ l , j is the twist angle of an SRR with respect to R C , where the first index reflects the number of SRR pair, and the second index distinguishes between the upper ( j =1) and lower ( j =2) SRRs in the pair. The dashed lines are the axes of mirror symmetry. ( c ) Schematic showing the phase transition of net chirality of the system when the incident power changes. In the shaded regime, spontaneous chiral symmetry breaking occurs and the net chirality can fall into either the left-handed (LH) or the right-handed (RH) regime. Full size image In the following sections, we start with the simple case of a pair of enantiomeric meta-molecules and show that chiral symmetry breaking can exist due to intermolecular interaction. This process leads to the sudden occurrence of polarization rotation and localization, an analogy to the phase-transition effects. Then, we reveal the underlying mechanism by analysing the evolution of local stability of the system, showing the critical role of intermolecular interaction in creating new stable states with broken chiral symmetry. Furthermore, we perform a proof-of-concept microwave experiment to study the nonlinear behaviour of a pair of enantiomeric meta-molecules, and the results provide a concrete verification of our theoretical prediction. Finally, we extend our study to meta-molecular necklaces with C N v symmetry and periodic arrays that mimic the situation in bulk torsional metamaterials. Our study demonstrates the possibility for creating artificial phase-change metamaterials via spontaneous chiral symmetry breaking. Coupled torsional meta-molecules with chiral symmetry The system studied is shown in Fig. 1 , with each torsional meta-molecule consisting of two coaxial split ring resonators (SRRs) connected by an elastic thin wire. We choose the radii of thin SRRs as r a =6 mm, slit width 1 mm and inter-ring distance 3 mm, the same as the configuration studied before [45] . For clarity, we denote the upper and lower SRRs of meta-molecule number l as ( l , 1) and ( l , 2), respectively. In the calculations, we fix the upper rings and restrict the allowed movement of the bottom rings to azimuthal rotation, while movement in the lateral and axial directions is usually negligible in comparison, and can be explicitly suppressed by the design if required [42] . For simplicity, we use a perfect electric conductor as the material for the SRRs in the simulation, so only the radiative component of the EM force is taken into account. To confirm the chiral symmetry of the system, 2 N ( NεN ) torsional meta-molecules with opposite handedness are symmetrically coupled and uniformly excited with the same amplitude and phase. For a finite system, this can be done by arranging the 2 N torsional meta-molecules in a way that the whole system satisfies C N v symmetry, that is, σ = π / N . The displacement vector pointing from the rotation centre O to the centre of a meta-molecule is R C , and θ is the twist angle of an SRR, defined by the orientation of the slit with respect to R C . We employ the following coupled equations to study the nonlinear response of the system (see Supplementary Methods for full details): Equation (1) is the set of coupled equations describing EM interactions, where Z is the effective impedance that depends on twist angles and separation, Q is the mode amplitude of oscillating current in the SRRs and is the electromotive force induced by the external fields. Equation (2) describes the torsional motion of the lower SRRs ( l , 2), where I is the moment of inertia and is the total torque experienced by the lower SRR. When the system is excited by an external wave, the twist angle θ l ,2 changes to a new stable position where the EM torque M EM and restoring torque from the elastic wire M R are balanced; this in turn changes the overall coupling Z as well as the EM response Q , and again the total torque. Owing to the resonant nature of the EM torque, such feedback can give rise to highly nonlinear effects, which can be found by solving Equation (1) and Equation (2) simultaneously. We start with the simplest case when two enantiomeric torsional meta-molecules are coupled. Without loss of generality, we choose the y – z plane as the plane of mirror symmetry and the system is excited with an x -polarized plane wave propagating in z direction, as shown in Fig. 1b . Since the Hamiltonian possesses chiral symmetry—the effective impedance Z has components Z (1,1),(2,2) = Z (2,1),(1,2) —the resulting mode amplitudes and EM torques also possess the same symmetry, that is, | Q 1,1 |=| Q 2,1 |, | Q 1,2 |=| Q 2,2 |, . As an example, we calculate the EM torque experienced by SRRs (1, 2) and (2, 2) (denoted as and ), with twist angles θ 1,1 =− θ 2,1 =90° and θ 1,2 =− θ 2,2 =45°, and | R C |=2.5 r a . It should be noted that, in a system with 2 N resonators, 2 N hybrid resonances can be supported in general. However, the number of resonances excited can be reduced due to symmetry. If the system satisfies C N v symmetry and is excited uniformly, only two resonances can be observed. This property provides an important spectral reference to estimate the chiral symmetry of the system in experiments. Since the EM interaction is dominated by the intramolecular coupling for such separation, the overall lineshape is qualitatively similar to a single meta-molecule. As can be seen from Fig. 2a , the directions of resonance-enhanced EM torques induced by the two hybrid modes are opposite due to the different mode symmetries [42] . 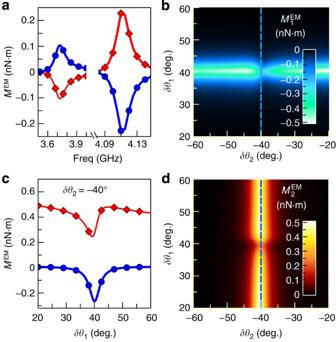Figure 2: EM torque experienced by the rotatable SRRs. (a) Spectra of EM torque experienced by SRRs (1,2) and (2,2) (denoted as(blue circles) and(red diamonds)), with twist anglesθ1,1=−θ2,1=90°,θ1,2=−θ2,2=45° and |RC|=2.5ra. (b) and (d) are the EM torque as functions of the two mutual twist anglesδθ1=θ1,1−θ1,2andδθ2=θ2,1−θ2,2, with pump frequency 4.1 GHz; the corresponding cross-sections along the blue dashed lines are shown in (c) (blue circles forand red diamonds for). The EM torque has been normalized to the power density of 1 mW mm−2. Figure 2: EM torque experienced by the rotatable SRRs. ( a ) Spectra of EM torque experienced by SRRs (1,2) and (2,2) (denoted as (blue circles) and (red diamonds)), with twist angles θ 1,1 =− θ 2,1 =90°, θ 1,2 =− θ 2,2 =45° and | R C |=2.5 r a . ( b ) and ( d ) are the EM torque as functions of the two mutual twist angles δθ 1 = θ 1,1 − θ 1,2 and δθ 2 = θ 2,1 − θ 2,2 , with pump frequency 4.1 GHz; the corresponding cross-sections along the blue dashed lines are shown in ( c ) (blue circles for and red diamonds for ). The EM torque has been normalized to the power density of 1 mW mm −2 . Full size image However, even a relatively weak intermolecular interaction is sufficient to introduce modulation of the resonant amplitude and of the EM torque. This effect can be clearly observed in Fig. 2b,d , which show the EM torques experienced by SRRs (1, 2) and (2, 2) under pump frequency 4.1 GHz as functions of the mutual twist angles ( δθ l = θ l ,1 − θ l ,2 ) in two meta-molecules. This modulation becomes the strongest when both meta-molecules are in resonance ( δθ 1 ≈− δθ 2 ) (see Fig. 2c for the cross-sections along the blue dashed lines). Note that although the EM torque experienced by a meta-molecule is still a Lorentz-like function of its own twist angle, it is also modulated by the twist angle from the other meta-molecule, which gives a more general Fano lineshape. Spontaneous chiral symmetry breaking in dimers As shown above, the interaction between two meta-molecules results in EM torque, which depends on the configuration of both meta-molecules. It is this interaction that modifies the stability of the system and leads to the spontaneous chiral symmetry breaking, as will be shown below. Importantly, such chiral symmetry breaking can be found in the stationary response of the system, which means this is an effect independent of mechanical damping, and this is a desirable property for their future realization in optics, since the promising fabrication approach based on DNA origami [48] requires a liquid environment. By calculating the dynamics of the system in Fig. 1 under different pump frequencies and power densities P I , we notice that such an effect can be found at frequencies just below resonance. For clarity, we focus on the resonance centred around 4.11 GHz, in which the currents of the two SRRs within each meta-molecule flow in opposite directions. For each frequency, the pump power density P I is increased from 0 to 4 mW mm −2 and decreased back to 0 mW mm −2 in steps of 0.05 mW mm −2 . The damping coefficient Γ=1.42 Hz is equivalent to the damping experienced in water, and the system can become stable after damped oscillations. The regime of broken symmetry can be found by summing the two stable twist angles, | δθ 1 + δθ 2 |, which would be non-zero if the symmetry is broken. The results clearly show that this symmetry breaking effect has hysteretic features (see Fig. 3a ). 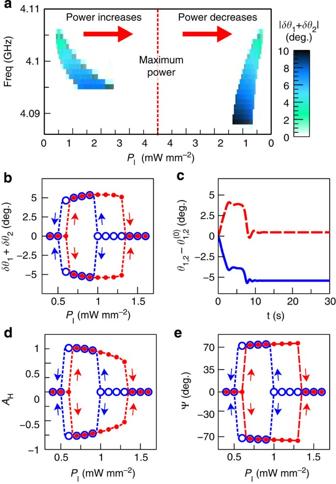Figure 3: Chiral symmetry breaking of enantiomeric dimers. (a) Regime of spontaneous chiral symmetry breaking as a function of incident power densityPIand pump frequency. The initial twist angles are chosen to be the same as inFig. 2. For pump frequency 4.10 GHz, (b) the asymmetry of twist angles, characterized byδθ1+δθ2, and (c) the corresponding time-dependent response of the symmetry-breaking process atPI=0.7 mW mm−2, whereare the initial twist angles; the blue solid curve and red dashed curve correspond toand, respectively. (d) The asymmetry of EM energy stored within each meta-molecule, and (e) the corresponding polarization rotation Ψ of the forward scattered wave. The red solid and blue empty circles denote the states under increasing and decreasing power, respectively. In the chiral symmetry broken regime, the system could fall into either state with opposite handedness. Figure 3: Chiral symmetry breaking of enantiomeric dimers. ( a ) Regime of spontaneous chiral symmetry breaking as a function of incident power density P I and pump frequency. The initial twist angles are chosen to be the same as in Fig. 2 . For pump frequency 4.10 GHz, ( b ) the asymmetry of twist angles, characterized by δθ 1 + δθ 2 , and ( c ) the corresponding time-dependent response of the symmetry-breaking process at P I =0.7 mW mm −2 , where are the initial twist angles; the blue solid curve and red dashed curve correspond to and , respectively. ( d ) The asymmetry of EM energy stored within each meta-molecule, and ( e ) the corresponding polarization rotation Ψ of the forward scattered wave. The red solid and blue empty circles denote the states under increasing and decreasing power, respectively. In the chiral symmetry broken regime, the system could fall into either state with opposite handedness. Full size image As an example, Fig. 3b depicts this process for a pump frequency of 4.1 GHz. The chiral symmetry of the system is preserved for low power. However, such symmetry can suddenly be broken ( δθ 1 + δθ 2 ≠0) when the pump power surpasses a certain threshold, and Fig. 3c depicts the dynamics of the lower rings (1, 2) and (2, 2) at the threshold power of 0.7 mW mm −2 , during which the system evolves from a symmetric state to an asymmetric state. The threshold powers can be different for increasing (red solid circles) and decreasing (blue open circles) power levels, showing hysteresis. At the threshold power level where chiral symmetry is broken, the system can fall from the symmetric state into either of the two asymmetric states with opposite handedness, and the final ‘observed’ state is random if there is no predefined bias in the initial state. This process is also known as ‘hidden’ symmetry [1] , [2] , since the two asymmetric states are still mirror symmetric with respect to each other, although only one of them can be finally ‘observed’ each time. In the near field, such broken symmetry directly leads to asymmetry of the EM energy confined by the torsional meta-molecules. Figure 3d depicts such a change, where the asymmetry factor is defined as A H =( H 1 − H 2 )/( H 1 + H 2 ), with being the energy confined in each meta-molecule. The most noticeable consequence of this symmetry breaking is the sudden occurrence of giant polarization rotation of forward/backward scattered waves (see Fig. 3e ), and this phase-transition process could provide a new mechanism to construct artificial phase-change metamaterials without introducing any naturally occurring phase-change materials [49] , as will be further confirmed below. Underlying mechanism The mechanism of the above process can be fully understood by analysing the local stability of the system. Figures 4a–c demonstrate how the total torque and equilibria evolve as pump power changes. The colour scale and vectors show the amplitude and direction of the total torque experienced by the system, and it is defined as . The blue and red curves correspond to M 1 =0 and M 2 =0, respectively; their crossovers are the equilibria of the system | M |=0, which is pump power-dependent. The local stability of the equilibria can be analysed by calculating the eigenvalues of the linearized dynamic equations [45] , [50] . Importantly, one can also evaluate the stability of the equilibria in Fig. 4 by identifying the direction of the vectors, which shows the direction of the total torque and tells whether an equilibrium is ‘attractive’ (stable) or ‘repulsive’ (unstable). 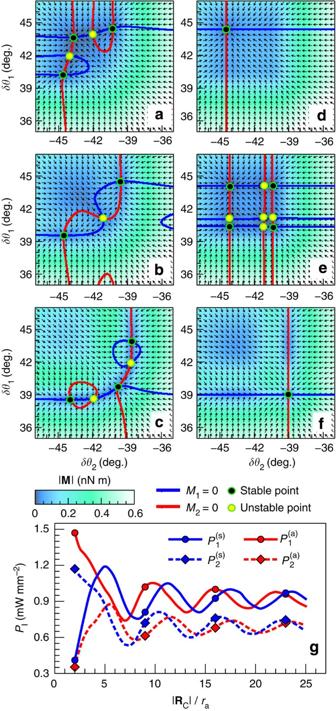Figure 4: Evolution of total torques and the threshold powers of bifurcation. (a–f) Total torque experienced by the system, under different pump power densities and intermolecular distances. The vectors and colour scale indicate the direction and amplitude of total torque, respectively. The crossovers ofM1=0 (blue curves) andM2=0 (red curves) are the equilibria of the system. (a,d) 0.55 mW mm−2, (b,e) 0.7 mW mm−2, (c,f) 1.2 mW mm−2. Pump frequency is 4.1 GHz, the same as inFig. 3b–e; |RC|=2.5rafor (a–c), and |RC|=250rafor (d–f). (g) Threshold powers of bifurcation for the two symmetric states (denoted as) and the asymmetric state (denoted as), as a function of |RC|. Figure 4: Evolution of total torques and the threshold powers of bifurcation. ( a – f ) Total torque experienced by the system , under different pump power densities and intermolecular distances. The vectors and colour scale indicate the direction and amplitude of total torque, respectively. The crossovers of M 1 =0 (blue curves) and M 2 =0 (red curves) are the equilibria of the system. ( a , d ) 0.55 mW mm −2 , ( b , e ) 0.7 mW mm −2 , ( c , f ) 1.2 mW mm −2 . Pump frequency is 4.1 GHz, the same as in Fig. 3b–e ; | R C |=2.5 r a for ( a – c ), and | R C |=250 r a for ( d – f ). ( g ) Threshold powers of bifurcation for the two symmetric states (denoted as ) and the asymmetric state (denoted as ), as a function of | R C |. Full size image As is shown in Fig. 4a , the stable equilibrium (black circle) of the symmetric state around δθ 1 =− δθ 2 ≈43.5° starts to overlap with the two unstable ones nearby (yellow circles), and it turns into an unstable point (undergoes a bifurcation) as power increases (see Fig. 4b ). Then the original symmetric state is no longer stable, and the system falls into either of the two nearby stable states by breaking the original chiral symmetry, as depicted in Fig. 4b,c . This asymmetric state exists below the second bifurcation threshold (see Fig. 4c , the stable points of asymmetric states overlap with the nearby unstable ones and disappear as power further increases), and the system hops back to the second stable symmetric state when the power density surpasses 1.3 mW mm −2 , as shown in Fig. 3b–e (see Supplementary Fig. 3 for more details). It has to be emphasized that the chiral symmetry breaking effect shown here is attributed to the EM interaction between meta-molecules. As shown in Fig. 2 , such interaction leads to additional modulation of the EM torques, and it directly results in different threshold powers of bifurcation for symmetric and asymmetric states, which provides a necessary (but not sufficient) condition for symmetry breaking. For simplicity, we denote by and the threshold powers of the two symmetric states under low and high pumping power density, and and are the threshold powers of the asymmetric state in the intermediate power regime. Figure 4g depicts the threshold powers of bifurcation for the symmetric and the asymmetric states as a function of | R C | under frequency 4.1 GHz. The threshold powers of bifurcation exhibit interesting asymptotically oscillating features due to the influence of retardation on the EM coupling. Note that for a given | R C |, the chiral symmetry breaking effects for increasing power and decreasing power only exist within the power regime of and , respectively. Thus the regime of symmetry breaking also follows similar asymptotically oscillating behaviour as | R C | increases. The oscillation period is the resonant wavelength in vacuum (for 4.1 GHz, the period is approximately 6 r a ), and the power regime of chiral symmetry breaking decreases dramatically as intermolecular separation enters the far-field regime (| R C |>6 r a ). Strictly speaking, the sufficient condition for chiral symmetry breaking is that when the bifurcation of one stable symmetric state happens, the only available state is the stable asymmetric state. The first situation that satisfies such sufficient condition is the case shown in Fig. 4a,b —when the bifurcation of the first symmetric state occurs, the second symmetric state has not emerged due to its higher threshold power of bifurcation , and the system can only fall into the existing asymmetric state. The second situation is such that when the bifurcation of the first symmetric state occurs the second symmetric state already exists ; however, due to an additional unstable point in between the two symmetric states (see the case of | R C |=4 r a in Supplementary Fig. 4 ), the trajectory of the system will still be ‘pushed’ away from the axis of δθ 1 =− δθ 2 and fall into the asymmetric state. The powers of bifurcation for symmetric and asymmetric states become degenerate eventually when the separation becomes very large. Figures 4d–f show the extreme situations under the same power densities as Figs 4a–c , but with very large distance | R C |=250 r a , at which the intermolecular interaction becomes negligible. As a result, the curves for M 1 =0 and M 2 =0 reduce to straight lines, and the stable points of the symmetric and asymmetric states around δθ 1 ≈44° and δθ 2 ≈−44° ( Fig. 4e ) will disappear simultaneously when the power further increases, since they have the same threshold power of bifurcation. In this case, the system can only jump to the second stable symmetric state with smaller mutual twist angles (see Fig. 4f ): this process is exactly the bistable hopping found in our previous study [42] . In contrast, the hysteresis shown in Fig. 3 is actually a multistable process, during which three independent stable states (two symmetric states for low and high power density, and one asymmetric state for intermediate power density) are accessed. Therefore, intermolecular interaction is indispensable for the existence of a non-degenerate state with broken chiral symmetry. Experimental verification We confirm the theoretical prediction of spontaneous chiral symmetry breaking by performing a pump-probe experiment in the microwave regime, with setup similar to that in ref. 42 . We have used four copper split-ring resonators printed on Rogers R4003 substrate to construct two pairs of chiral meta-molecules. The outer radius, track width, slit width and thickness of each SRR are 4.2, 1.0, 0.2 and 0.035 mm, respectively. Two of the SRRs are fixed on a polystyrene block and positioned at the centre of a circular waveguide, with their slits oriented parallel to the wave propagation direction (see Fig. 5 ). The other two SRRs are suspended with thin rubber wires (radius a =50 μm, length d =19.4 mm and shear modulus 0.6 MPa), and are well aligned coaxially with the two fixed SRRs, with a face-to-face distance of ~1.2 mm and the initial twist angles . The centre–centre distance of the two chiral meta-molecules is 12.7 mm. Due to experimental constraints, the orientation of the incident field relative to the meta-molecules differs from that in our theoretical analysis; however, by exciting the two meta-molecules with the same magnitude and phase, we preserve the symmetry required to demonstrate the effect. The two pairs of twisted split rings are positioned in a circular waveguide, and are excited with the TE 11 waveguide mode, having its electric field parallel to the SRRs. 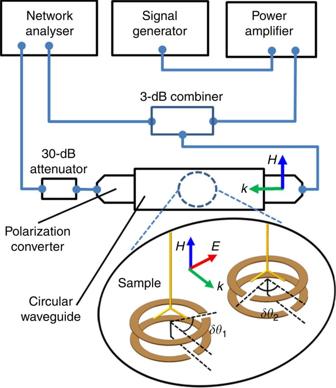Figure 5: Experimental setup. Schematic of the experimental setup of microwave pump-probe measurement. For clarity, the substrate of the sample is omitted. Figure 5: Experimental setup. Schematic of the experimental setup of microwave pump-probe measurement. For clarity, the substrate of the sample is omitted. Full size image The transmission spectrum is measured by a vector network analyser (Rohde and Schwarz ZVB-20). In general, the four-SRR system can give rise to four resonances due to mutual coupling, and two of them can be observed within the frequency regime of interest (<4 GHz). These two modes can be understood as a further hybridization of the original symmetric modes (with currents flowing in the same direction) supported by the SRR pairs, as discussed in our previous studies [42] , [51] . However, in the chiral symmetric configuration, one of these two modes will not be excited due to its zero overlap with the incident field. This property provides an accurate reference for tuning the initial positions of the two twisted SRR pairs—only when the two ring pairs are positioned almost perfectly symmetrically can we observe a single resonance with Lorentz lineshape. Our simulation further confirms that the ‘hidden’ mode can be excited and becomes easily distinguishable once the difference of initial twist angles becomes larger than 1°. Thus, the horizontal positions, the longitudinal separations and the initial twist angles can be carefully adjusted so that only one resonance is observed. We choose a pump frequency of 3.53 GHz, which is just below the initial resonance of ~3.55 GHz. The CW pump signal is generated by a signal generator (HP 8673B) and is further amplified by a power amplifier (ZHL-16W-43-S+). The pump power is increased in steps of 0.5 dB and the spectra are recorded once the system reaches a steady state. The normalized transmission spectra | S 21 | as a function of pump power are plotted in Fig. 6a , where the black dots denote the positions of the resonances, and the blank regime is where the system undergoes self-oscillations, hence no steady-state signal can be recorded. It is clearly shown that the original single resonance at ~3.55 GHz red shifts as pump power increases, and it suddenly splits into two new resonances when the power surpasses 24 dBm. This is clear evidence for the existence of spontaneous chiral symmetry breaking. 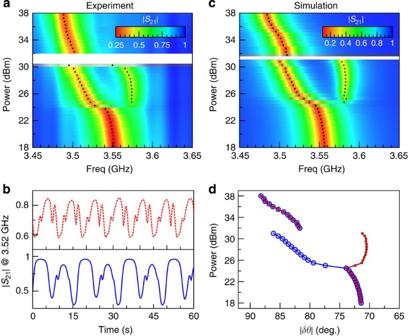Figure 6: Observation of chiral symmetry breaking and self-oscillation. (a) Measured transmission spectra in stationary state as a function of pump power. The pump frequency is chosen at 3.53 GHz, and the power is swept from 18 to 38 dBm in 0.5 dB steps. The black dots denote the position of the resonances, and the blank area shows region of parameters where self-oscillation occurs. (b) Time evolution of transmission coefficient at 3.52 GHz when the system exhibits self-oscillation. The red dashed curve and blue solid curve correspond to pump power 30.5 and 31 dBm, respectively. (c) Simulated transmission spectra and (d) the corresponding fitted mutual twist angles for different power levels, where red solid circles and blue open circles correspond to |δθ1| and |δθ2|, respectively. Figure 6: Observation of chiral symmetry breaking and self-oscillation. ( a ) Measured transmission spectra in stationary state as a function of pump power. The pump frequency is chosen at 3.53 GHz, and the power is swept from 18 to 38 dBm in 0.5 dB steps. The black dots denote the position of the resonances, and the blank area shows region of parameters where self-oscillation occurs. ( b ) Time evolution of transmission coefficient at 3.52 GHz when the system exhibits self-oscillation. The red dashed curve and blue solid curve correspond to pump power 30.5 and 31 dBm, respectively. ( c ) Simulated transmission spectra and ( d ) the corresponding fitted mutual twist angles for different power levels, where red solid circles and blue open circles correspond to | δθ 1 | and | δθ 2 |, respectively. Full size image As the power further increases, the state with broken symmetry becomes unstable and the system exhibits self-oscillations. This effect is mainly due to the absence of stable state in the system [45] . We choose a probe frequency of 3.52 GHz to record the time evolution of the transmission coefficient. Some of the examples are shown in Fig. 6b , where the periodicity of the signals indicates that the system undergoes limit cycles. For other pump powers, more complicated behaviour such as aperiodic or even chaos-like trajectories is observed ( Supplementary Fig. 5 ). Remarkably, the system becomes stable again when the power exceeds 32 dBm. The two split resonances disappear and a new single resonance appears at ~3.5 GHz, which red shifts as power further increases. This is a clear verification of our theoretical prediction that the system will eventually hop back to the second symmetric state (the only stable state) when the pump power is sufficiently strong. Finally, we perform full-wave simulation using CST Microwave Studio to reproduce the measured spectra by taking into account the influence of substrate and waveguide. We calculate the EM torque experienced by the two suspended SRRs under different mutual twist angles ( δθ 1 , δθ 2 ) when the structure is pumped at frequency 3.53 GHz, and the result gives a two-dimensional map similar to Fig. 2b,d . Then the equilibria of the system and their stability under different pump power can be found by following the procedure used in Fig. 4 , in which the initial twist angles are chosen as δθ 1 =− δθ 2 =71°. These stable mutual twist angles can again be remapped to the transmission spectra. The transmission coefficients under different pump power and the corresponding stable mutual twist angles are shown in Fig. 6c,d (for clarity, we only plot one of the possible asymmetric states where | δθ 1 |<| δθ 2 |). Despite the complexity of the system, the simulation spectra are in good agreement with the measured results. As can be seen, in the power regime where chiral symmetry breaking happens (| δθ 1 |≠| δθ 2 |), the original single resonance splits into two; it is also confirmed by the stability analysis that the system does not possess any stable equilibrium in the blank regime, which leads to self-oscillations. Therefore, the evolution of chiral symmetry breaking predicted above—from the symmetric state at low pump power to an asymmetric state in the intermediate power regime, and finally back to the symmetric state at high power—is fully verified by the experiment. Enantiomeric necklace rings and arrays Having revealed the basic mechanism of chiral symmetry breaking in dimer enantiomers, it is desirable to show how this mechanism can influence the behaviour in larger-scale systems where more than two enantiomers are coupled, and to determine whether this process can be applied to realize phase-change metamaterials. To do so, we extend our theoretical study of dimer enantiomers to more complex systems. One very interesting configuration is a necklace ring composed of 2 N enantiomeric meta-molecules with the configuration of the whole system satisfying C N v symmetry, as shown in Fig. 1b . To excite all the meta-molecules uniformly, one can use azimuthally polarized waves. In the following calculation, we use the same initial twist angles and for all the necklace rings, and the radius of necklace | R C | is chosen such that the centre–centre distance between nearest-neighbouring meta-molecules is 5 r a . By calculating the dynamic and stable states of the system, we notice that despite the complexity of nonlinear modes available, these modes still satisfy the same symmetry as the structure. Similar to the dimer enantiomers, the system always occupies the C N v states under low or high power density, in which the system has only one stable point. In the intermediate power level where more than one stable point can exist, various states with reduced symmetry are available, including those with broken mirror symmetry (such as C N states), reduced rotational symmetry ( C n v | n < N states) and completely broken symmetry ( C 1 states). Within these various types of nonlinear states, the C N | N >2 states are particularly interesting, since structures with such symmetry are intrinsically isotropic and their corresponding eigenstates of forward/backward radiation are circular polarized. Some examples of these modes are shown in Fig. 7a , in which the direction of the rotation angle is indicated by red open circles and blue solid circles, and its magnitude is represented by the distance between the circle and the centre of the polar plot. 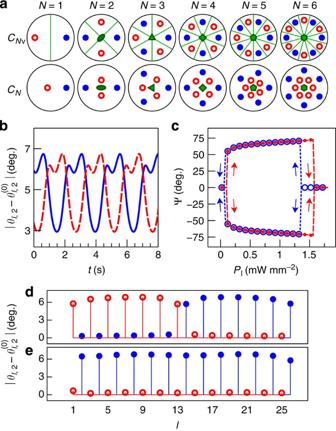Figure 7: Chiral symmetry breaking in necklace rings and 1D arrays. (a) Examples of nonlinear modes withCNvandCNsymmetry accessed by the necklace rings with 2Nenantiomeric meta-molecules. The direction of angle rotation of SRRs is denoted with red open circlesand blue solid circles; the distance between the circle and the centre of polar plots denotes the magnitude of rotation. (b) Time evolution of self-oscillation states for the necklace withC5symmetry. The pump frequency and power density are 4.105 GHz and 1.8 mW mm−2, respectively. The blue solid curve and red dashed curve correspond to the dynamics of SRRs withand, respectively. (c) Polarization rotation of forward scattered waves in an infinite array of enantiomeric meta-molecules, as a function of pump power density; pump frequency is chosen as 4.1 GHz for comparison withFig. 3e. An example of chiral symmetry breaking in a finite 1D array (13 enantiomeric pairs) with (d) a symmetric excitation, and (e) a small perturbation in polarization (0.05°). The configuration of meta-molecules and the periodicity are the same as the infinite array. The frequency and power density are 4.1 GHz and 0.8 mW mm−2, respectively. Figure 7: Chiral symmetry breaking in necklace rings and 1D arrays. ( a ) Examples of nonlinear modes with C N v and C N symmetry accessed by the necklace rings with 2 N enantiomeric meta-molecules. The direction of angle rotation of SRRs is denoted with red open circles and blue solid circles ; the distance between the circle and the centre of polar plots denotes the magnitude of rotation. ( b ) Time evolution of self-oscillation states for the necklace with C 5 symmetry. The pump frequency and power density are 4.105 GHz and 1.8 mW mm −2 , respectively. The blue solid curve and red dashed curve correspond to the dynamics of SRRs with and , respectively. ( c ) Polarization rotation of forward scattered waves in an infinite array of enantiomeric meta-molecules, as a function of pump power density; pump frequency is chosen as 4.1 GHz for comparison with Fig. 3e . An example of chiral symmetry breaking in a finite 1D array (13 enantiomeric pairs) with ( d ) a symmetric excitation, and ( e ) a small perturbation in polarization (0.05°). The configuration of meta-molecules and the periodicity are the same as the infinite array. The frequency and power density are 4.1 GHz and 0.8 mW mm −2 , respectively. Full size image Another exotic type of behaviour that the necklace ring can also exhibit is self-oscillations. These occur when the system has no stable point and enters a consistent oscillation state, corresponding to the limit cycle on the phase diagram. This mechanism is the same as what we discovered recently and thus the oscillations are damping-immune [45] . Interestingly, some of these oscillation states still satisfy C N symmetry, and an example of N =5 is depicted in Fig. 7b , which shows the time evolution of the rotation angles of SRRs ( l , 2). Remarkably, due to the chiral symmetry of the system, the oscillation amplitudes of meta-molecules with and are exactly the same; this means the system actually oscillates back and forth between the unstable left-handed and right-handed C N states—the ‘hidden’ symmetry of the system is revealed via self-oscillations. Finally, we study the phase transition in an array of enantiomeric meta-molecules. We first calculate the response of a one-dimensional infinite array to check the feasibility of the effect. We employ periodic boundary conditions to simplify the problem, assuming that the EM and mechanical responses in all the unit cells are identical, and the degree of freedom of the whole system can be reduced to 2. By taking into account the coupling of over 360 neighbouring meta-molecules in the multipole expansion model (see Supplementary Methods ), the results converge. For convenience of comparison, we depict the polarization rotation of forward scattered wave of an array in Fig. 7c . The unit cell of the array is a pair of enantiomeric dimers ( Fig. 1b ), with configuration the same as the one studied in Fig. 3 ; the pump frequency and the incident polarization (along x direction) are also identical to the case shown in Fig. 3e . The array is periodic along the x direction, with a periodicity of 10 r a . Despite the more complex and long-range coupling in an infinite array, the overall behaviour is still similar to that shown for dimers, since the origin of symmetry breaking in our system is intermolecular interaction. As can be seen, the chiral symmetry is preserved for low and high power, and such symmetry is broken within some intermediate power regime, which leads to the existence of giant polarization rotation. The power regime of symmetry breaking becomes wider than the case of a dimer (see Fig. 3e ) due to the stronger intermolecular interaction in the array system. We note that the periodic boundary condition used above is a simplification that neglects many other possible solutions of symmetry breaking. In general, the nonlinear behaviour of an array system, with either finite or infinite size, can be very complicated if the number of degrees of freedom is large, and the spontaneous chiral symmetry breaking effect would occur in the form of domains, as in many natural materials. However, by properly engineering our artificial materials, it is technically possible to exclude the undesirable complexity and achieve uniform chiral response over the whole system. One simple concept is to mechanically connect all the meta-molecules of the same handedness, so that all the left-handed or right-handed meta-molecules can have identical deformation and the degree of freedom of the whole system can be reduced to 2 (for conceptual layouts of 2D array, see Supplementary Fig. 6 ). Alternatively, it is also possible to access uniform chiral response by introducing a small perturbation in the polarization state of incident waves, so that the left-handed and right-handed meta-molecules experience a slightly different EM torque. Such variation has little influence when the system is operated in the linear regime, but it can be used to control the symmetry breaking effect, since the system is highly sensitive to small perturbations around critical points. Figures 7d,e show an example of the chiral symmetry breaking response of a 1D finite array (13 enantiomeric pairs) under the same pump frequency and power density, but with slightly different polarization states. The configuration of meta-molecules, the periodicity and the pump frequency are the same as those of the infinite array. As can be seen, under the same pump power density, the original chiral domain response under symmetric excitation (polarization in x direction) turns into uniform chiral response when a small perturbation (0.05°) is introduced. A further study of the complex behaviour is beyond the scope of this paper. Therefore, the chiral symmetry breaking effect for the necklace and array systems shown above can be considered as a chiral analogy of the phase transition from the anti-ferromagnetic state to the ferrimagnetic state found in iron selenide [52] , [53] , and it shows a new possibility to create and design artificial phase-transition effects on demand in metamaterials, without the need of introducing naturally existing phase-change materials. We introduced and developed the concept of spontaneous chiral symmetry breaking in metamaterials. We studied the nonlinear behaviour of coupled enantiomeric torsional meta-molecules and revealed that such a structure leads to a variety of novel effects in the physics of metamaterials. In particular, we demonstrated that when the intermolecular coupling becomes sufficiently strong the system can exhibit a phase transition by suddenly breaking the original chiral symmetry. We studied the underlying mechanism of this effect and analysed the evolution of the system stability, revealing that intermolecular interaction is indispensable for the existence of asymmetric states. We explored such processes in enantiomeric necklace rings and infinite arrays of meta-molecules, showing that spontaneous chiral symmetry breaking provides a novel and feasible mechanism for creating artificial phase transitions in assemblies of meta-molecules without naturally occurring phase-change materials. To verify the feasibility of our concept, we performed a pump-probe microwave experiment, and the results provide a concrete verification of our theoretical predictions. Although the study here is based on torsional structures, it is expected that a similar effect would also exist in other structures that are easier to fabricate, such as cantilevers and beams that can support bistable or multistable responses induced by EM-elastic (or opto-mechanical) coupling. Given the developments of fabrication technologies, this artificial phase-change effect should be observable in metamaterials and meta-surfaces for a wide variety of wavelength ranges. The critical phenomena around the bifurcation points may reveal yet further interesting phenomena, since, unlike most of its analogies in condensed-matter systems, the system studied here is non-conservative. The possibility of using such instability around the critical points for ultra-high sensitive measurements is quite exciting. Furthermore, the achiral–chiral transition shown here is not the only one possible in metamaterials; there are also positive–negative index and elliptic–hyperbolic dispersion transitions that warrant exploration. How to cite this article: Liu, M. et al. Spontaneous chiral symmetry breaking in metamaterials. Nat. Commun. 5:4441 doi: 10.1038/ncomms5441 (2014).